A highly efficient polysulfide mediator for lithium–sulfur batteries The lithium–sulfur battery is receiving intense interest because its theoretical energy density exceeds that of lithium-ion batteries at much lower cost, but practical applications are still hindered by capacity decay caused by the polysulfide shuttle. Here we report a strategy to entrap polysulfides in the cathode that relies on a chemical process, whereby a host—manganese dioxide nanosheets serve as the prototype—reacts with initially formed lithium polysulfides to form surface-bound intermediates. These function as a redox shuttle to catenate and bind ‘higher’ polysulfides, and convert them on reduction to insoluble lithium sulfide via disproportionation. The sulfur/manganese dioxide nanosheet composite with 75 wt% sulfur exhibits a reversible capacity of 1,300 mA h g −1 at moderate rates and a fade rate over 2,000 cycles of 0.036%/cycle, among the best reported to date. We furthermore show that this mechanism extends to graphene oxide and suggest it can be employed more widely. As the development of portable electronics devices, electric vehicles and large-scale energy storage increases, so do the demands for energy storage batteries with high energy density and long service life. At the same time, it is recognized that traditional lithium-ion batteries are approaching their theoretical energy density limits [1] , [2] , [3] , [4] . Lithium–sulfur batteries are one of the most promising candidates to satisfy emerging market demands [5] , [6] , [7] , as they possess a theoretical capacity and energy density of 1,675 mA h g −1 and 2,500 kW kg −1 , respectively, superior to current lithium-ion batteries [8] , [9] . In addition, they present an inherently low competitive cost due to the high natural abundance of sulfur. These advantages suggest that the lithium–sulfur battery should be capable of energy storage several times greater than conventional lithium-ion batteries, with reduced cost. However, practical applications are currently hindered by several obstacles. These predominantly relate to the insulating nature of sulfur and lithium sulfides, which require addition of conductive additives (hence lowering the active sulfur mass fraction), pronounced capacity fading on cycling and an internal redox shuttle that lowers Coulombic efficiency [10] . Over decades, much effort has been expended to try to solve these problems by trapping the polysulfides within the cathode structure. The most popular approaches are to encapsulate sulfur in the pores of carbon materials or a conductive polymer matrix. Meso/microporous carbons [11] , [12] , [13] , [14] , carbon spheres [15] , [16] , [17] , carbon nanotubes/fibres [18] , [19] , [20] , polyaniline [21] , polypyrrole [22] , [23] and poly(3,4-ethylenedioxythiophene) [24] sulfur-host cathodes have all had a positive effect on increasing the cycle life of lithium–sulfur cells. However, such architectures and polymer coatings can only partially retain polysulfides and are limited in their function over time, owing to structural changes that arise from the 80% volume change of the sulfur cathode on discharge. Two-dimensional materials such as graphene oxides (GOs) have also been very successfully employed as cathode hosts to increase the performance of the lithium–sulfur battery, where interaction between the oxygen/nitrogen functional groups and sulfur/polysulfides has been suggested [25] , [26] , [27] , [28] . Similarly, binding polysulfides onto hydrophilic metal oxide hosts was shown to significantly aid in maintaining high-capacity retention [29] , [30] , [31] . More recently, high-surface-area polar metallic oxides have been used as a two-in-one approach to provide both a ‘sulfiphilic’ surface and supply electron transport to effect surface-enhanced redox chemistry [32] ; or to spatially locate Li 2 S deposition and enhance redox [33] . Organometallic redox mediators are shown to provide better utilization of Li 2 S (ref. 34 ). Additives such as P 2 S 5 also effectively control Li 2 S deposition and aid in elimination of the polysulfide shuttle [35] . Herein, we present a quite different chemical approach to polysulfide retention in the sulfur cathode, which relies on mediating polysulfide redox through insoluble thiosulfate species in a two-step process. The thiosulfate groups are first created in situ by oxidation of initially formed soluble lithium polysulfide (LiPS) species on the surface of ultra-thin MnO 2 nanosheets. As reduction proceeds, the surface thiosulfate groups are proposed to anchor newly formed soluble ‘higher’ polysulfides by catenating them to form polythionates and converting them to insoluble ‘lower’ polysulfides. The polythionate complex formed on the surface is thus best described as a transfer mediator. This process curtails active mass loss during the discharge/charge process and supresses the polysulfide shuttle to result in high-performance cathodes with high sulfur loading, capable of high-capacity retention of 92% after 200 cycles at a C/5 rate and cycling over 2,000 cycles at 2C with a capacity decay of 0.036% per cycle. Synthesis and characterization The MnO 2 nanosheets were prepared by reducing GO with KMnO 4 (ref. 36 ). Transmission electron microscopy (TEM) and scanning electron microscopy (SEM) images ( Fig. 1a,b ) reveal their two-dimensional lamellar structure. The selected area electron diffraction pattern of the MnO 2 nanosheets shows weak diffraction rings characteristic of δ -MnO 2 , and the high-resolution TEM image in Fig. 1c exhibits a 0.25-nm lattice spacing corresponding to the (100) planes. X-ray diffraction ( Fig. 1d ) analysis confirms the MnO 2 nanosheets are monoclinic birnessite, δ -MnO 2 (JCPDS-01-080-1098). Birnessite is a phyllomanganate, a manganese oxide containing predominantly Mn 4+ cations assembled in layers of edge-sharing octahedra. A layer charge deficit arises from the presence of Mn 3+ cations and/or vacant-layer octahedra and is compensated by the presence of interlayer cations, which are hydrolysable K + in this case. Water molecules are also present between the sheets of MnO 6 octahedra, coordinated both to the Mn and the K, with some fraction of the former being present as hydroxyl groups [37] . Thermogravimetric analysis (TGA, Supplementary Fig. 1a ) reveals that the as-prepared MnO 2 nanosheets possess 8 wt% surface-absorbed water and 3 wt% water in the interlayers. Melt diffusion at 155 °C was used to uniformly disperse sulfur onto the surface of the MnO 2 nanosheets [28] , [29] , [30] . To maximize contact, the nanosheets were first pre-dispersed by sonication before being mixed with sulfur nanoparticles (see Methods) in a 25:75 weight ratio ( Supplementary Fig. 2 ). The TEM and SEM images in Fig. 1e,f show a homogeneous sulfur coating on the nanosheet surface after melt diffusion, as confirmed by energy dispersive X-ray spectroscopy mapping ( Supplementary Fig. 3 ). The targeted high sulfur loading of 75 wt% was achieved (TGA analysis of 75S/MnO 2 , Supplementary Fig. 1b ). 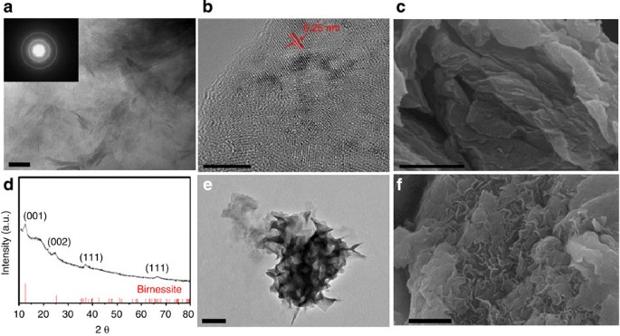Figure 1: Morphology and characteristics of the MnO2nanosheets and S/MnO2composite. (a) TEM image of MnO2nanosheets and its corresponding selected area electron diffraction pattern, (b) high-resolution TEM image of MnO2nanosheets, (c) SEM image of the MnO2nanosheets, (d) X-ray diffraction pattern of MnO2nanosheets, (e) TEM and (f) SEM images of the S/MnO2nanosheets composite. Scale bars, 50 nm (a); 100 nm (b,c,f); 200 nm (e). Figure 1: Morphology and characteristics of the MnO 2 nanosheets and S/MnO 2 composite. ( a ) TEM image of MnO 2 nanosheets and its corresponding selected area electron diffraction pattern, ( b ) high-resolution TEM image of MnO 2 nanosheets, ( c ) SEM image of the MnO 2 nanosheets, ( d ) X-ray diffraction pattern of MnO 2 nanosheets, ( e ) TEM and ( f ) SEM images of the S/MnO 2 nanosheets composite. Scale bars, 50 nm ( a ); 100 nm ( b , c , f ); 200 nm ( e ). Full size image Electrochemical properties Electrochemical behaviour evaluated at different current densities for the 75S/MnO 2 nanocomposite, showed characteristic Li-S voltage profiles ( Fig. 2a ) [12] , [14] . The cells exhibit a capacity of ~1,300 mA h g −1 at C/20 (discharge/charge of full theoretical capacity in 20 h). At a 20-fold higher current density (a C rate), only a modest drop in capacity to 950 mA h g −1 was observed, suggestive of highly efficient kinetics. Most notable is the lack of overpotential in the initial charging process even on the first cycle, indicative of a good Li 2 S interface with the MnO 2 nanosheets. 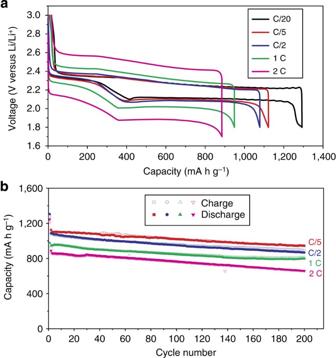Figure 2: Electrochemical performance of S/MnO2. (a) Voltage profiles of S/MnO2nanosheets at current densities ranging from C/20 to 2C. The highlighted circle shows the lack of overpotential. (b) Cycling performance of S/MnO2nanosheets at C/5, C/2, 1C and 2C rates. The cells were subjected to an initial slow conditioning cycle at C/20 to allow complete access of the electrolyte to the active material. Figure 2b shows the cycling stability of the cells at different rates. At C/5, the initial discharge capacity was 1,120 mA h g −1 , with 1,030 mA h g −1 being sustained after more than 200 cycles and representing excellent capacity retention of 0.04% per cycle. At higher current densities (1C), the 75S/MnO 2 composite still delivered exceptional reversible capacity of 800 mA h g −1 after 200 cycles. This indicates that processes such as loss of electrical contact of Li 2 S or sulfur with the conductive host caused by volume changes or the ‘shuttle reaction’ caused by the solubilized polysulfides are minimized. Figure 2: Electrochemical performance of S/MnO 2 . ( a ) Voltage profiles of S/MnO 2 nanosheets at current densities ranging from C/20 to 2C. The highlighted circle shows the lack of overpotential. ( b ) Cycling performance of S/MnO 2 nanosheets at C/5, C/2, 1C and 2C rates. The cells were subjected to an initial slow conditioning cycle at C/20 to allow complete access of the electrolyte to the active material. Full size image In-situ visual–electrochemical study of 75S/MnO 2 To further illustrate the excellent properties discussed above, we examined electrochemical behaviour of 75S/MnO 2 in an optically transparent Li–S cell, exploiting the very strong colour of LiPSs to probe their interaction with the cathode surface. Recent reports have visually demonstrated the binding of LiPSs with metallic metal oxide sulfur hosts such as Ti 4 O 7 (ref. 32 ) and spatially localized deposition of Li 2 S on conductive indium-tin oxide [33] . With δ -MnO 2 —a poor semiconductor—the interaction is based on a very different principle, as detailed in the next section. The cell using 75S/MnO 2 as the cathode clearly demonstrates the ability of the nanosheet host to control LiPS dissolution. For comparison, results are shown for a S/Ketjen Black (75S/KB) cathode prepared with the same 75% sulfur loading ( Fig. 3 ). 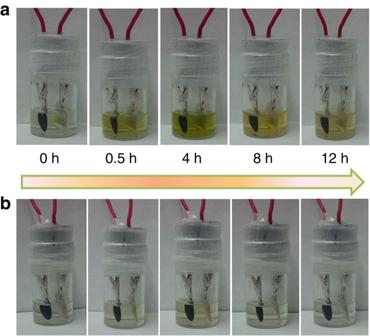Figure 3: Visual confirmation of polysulfide entrapment at specific discharge depths. (a) 75S/KB and (b) 75S/MnO2cells. These were both discharged at C/20 between open circuit potential to 1.8 V under identical conditions. Figure 3a reveals that the electrolyte in the 75S/KB cell changed from colourless to bright yellow–green on partial discharge of the cell over 4 h. This point corresponds to the ‘knee’ in the discharge curve at a capacity of 400 m Ah g −1 (a potential of 2.1 V, see Fig. 2a ), where the LiPS concentration is expected to be at a maximum. The characteristic colour of medium chain LiPSs (i.e, ~, S 4 2− ) indicates that the polysulfides diffuse out of the cathode and are solubilized in the electrolyte. Figure 3: Visual confirmation of polysulfide entrapment at specific discharge depths. ( a ) 75S/KB and ( b ) 75S/MnO 2 cells. These were both discharged at C/20 between open circuit potential to 1.8 V under identical conditions. Full size image At the end of discharge (12 h), the electrolyte is still yellow, showing LiPSs remain in solution. In contrast, in the 75S/MnO 2 cell the electrolyte exhibits only a faint yellow colour at 4 h. This provides striking visual evidence of very low LiPS content in the electrolyte and demonstrates effective trapping by the MnO 2 . On full discharge, the electrolyte is rendered completely colourless, indicating effective conversion to insoluble reduced species, Li 2 S 2 and Li 2 S. A test of the polysulfide adsorption by the MnO 2 nanosheets was conducted by electrochemical titration to measure the degree of residual LiPS in solution after contact, confirming the strong binding ( Supplementary Fig. 4 ) [38] . XPS study of the interaction of lithium (poly)sulfides and MnO 2 nanosheets The nature of the interaction of the MnO 2 nanosheets with LiPSs was determined from Mn 3 p 3/2 and S2 p X-ray photoelectron spectroscopy (XPS) analysis. Only the peak position of the lower binding energy component of the S2 p 3/2 /2 p 1/2 spin orbit doublet is described in the subsequent discussion following convention. The results are summarized in Figs 4 and 5 . 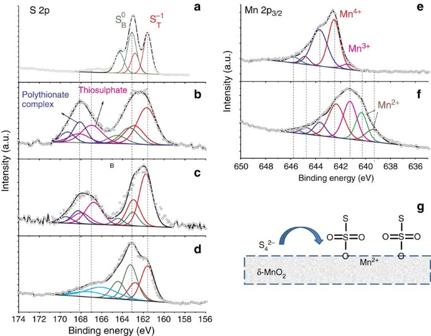Figure 4: XPS study of the interaction between sulfur species and MnO2nanosheets. S2pcore spectra of (a) Li2S4showing the terminal and bridging sulfur atoms in the expected 1:1 ratio; (b) MnO2-Li2S4and (c) GO–Li2S4exhibiting the thiosulfate/polythionate active groups and (d) ‘graphene’–Li2S4showing their absence; the contribution in turquoise is due to sulfite (from the Li2S4)32. Mn 2p3/2spectra of (e) MnO2nanosheets and (f) MnO2-Li2S4. (g) Schematic showing the oxidation of initially formed polysulphide byδ-MnO2to form thiosulfate on the surface, concomitant with the reduction of Mn4+to Mn2+. Figure 4: XPS study of the interaction between sulfur species and MnO 2 nanosheets. S2 p core spectra of ( a ) Li 2 S 4 showing the terminal and bridging sulfur atoms in the expected 1:1 ratio; ( b ) MnO 2 -Li 2 S 4 and ( c ) GO–Li 2 S 4 exhibiting the thiosulfate/polythionate active groups and ( d ) ‘graphene’–Li 2 S 4 showing their absence; the contribution in turquoise is due to sulfite (from the Li 2 S 4 ) [32] . Mn 2 p 3/2 spectra of ( e ) MnO 2 nanosheets and ( f ) MnO 2 -Li 2 S 4 . ( g ) Schematic showing the oxidation of initially formed polysulphide by δ -MnO 2 to form thiosulfate on the surface, concomitant with the reduction of Mn 4+ to Mn 2+ . 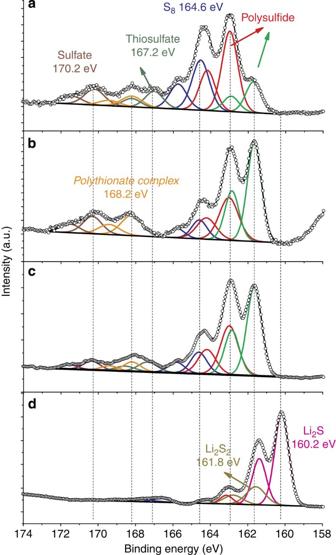Figure 5:Ex-situXPS of S/MnO2nanosheets electrodes after discharge to specific states. (a) Discharged to 2.15 V, (b) discharged to 2.15 V and then aged in the cell for 20 h, (c) discharged to 800 mA h g−1(the middle of the second plateau) and (d) discharged to 1.8 V. All cells were galvanostatically discharged at C/20 with 1 M LiClO4in DOL/DME (1:1 vol) as the electrolyte. The trace of sulfate at 170.2 eV is due to momentary air exposure during the XPS sample loading process. Full size image Figure 5: Ex-situ XPS of S/MnO 2 nanosheets electrodes after discharge to specific states. ( a ) Discharged to 2.15 V, ( b ) discharged to 2.15 V and then aged in the cell for 20 h, ( c ) discharged to 800 mA h g −1 (the middle of the second plateau) and ( d ) discharged to 1.8 V. All cells were galvanostatically discharged at C/20 with 1 M LiClO 4 in DOL/DME (1:1 vol) as the electrolyte. The trace of sulfate at 170.2 eV is due to momentary air exposure during the XPS sample loading process. Full size image Li 2 S 4 was employed as the representative polysulfide species to probe the system at a partial state of discharge. Its XPS spectrum ( Fig. 4a ) shows a 1:1 ratio of the two S2 p 3/2 contributions at 161.7 and 163.1 eV, ascribed to the terminal (S T −1 ) and bridging sulfur (S B 0 ) atoms, respectively. This assignment is in accord with the chain structure of Li 2 S 4 , where the sulfur atoms at both ends have a formal charge of (−1), while those in the middle bear a formal charge of (0) [32] , [39] . Figure 4e displays the XPS Mn 2p 3/2 spectra of δ -MnO 2 , which is mainly composed of Mn 4+ , with its near-surface enriched in Mn 3+ relative to the bulk [40] . The MnO 2 nanosheet spectrum is typical of birnessite [41] , showing a strong Mn 2 p 3/2 Mn 4+ contribution that appears as a characteristic multiplet with a maximum at 642.5 eV, and three satellite peaks at higher binding energies of 643.7, 644.8 and 645.7 eV. The ratio of the multiplet peaks is in agreement with calculations [41] . The Mn 2 p 3/2 contribution at 641.4 eV corresponds to Mn 3+ , which makes up ~4.6% of the MnO 2 nanosheets. To examine the LiPS–Mn interaction, a suspension of vacuum-dried δ -MnO 2 in ether was added to a solution of yellow–green Li 2 S 4 in dimethoxyethane, resulting in immediate discolouration. XPS data were collected on the recovered solid (‘MnO 2 –Li 2 S 4 ’). Its S2 p spectrum ( Fig. 4b ) reveals four sulfur environments. Two are the same terminal and bridging S environments as in Li 2 S 4 . The new significant contribution between 171 and 165 eV can be fit with two sulfur environments. The S2 p 3/2 peak at 167.2 eV is in precise accord with the binding energy of thiosulfate [42] , which must arise from a surface redox reaction between Li 2 S 4 and δ -MnO 2 . This peak is from the ‘central’ or S=O sulfur in thiosulfate ([SSO 3 ] 2− ), whereas its ‘peripheral’ sulfur lies at 161.5 eV, contributing to the S T −1 from residual Li 2 S 4 (thus accounting for the change in ratio of the (S T −1 :S B 0 ) 2 p 3/2 peaks from 1:1 to 2.4:1). The S2 p XPS spectrum of sodium thiosulfate is provided for reference ( Supplementary Fig. 5a ). The other S2 p 3/2 peak at 168.2 eV (ascribed to a polythionate complex in the MnO 2 –Li 2 S 4 material) will be discussed below. Oxidation of Li 2 S 4 to thiosulfate is accompanied by a decrease in the Mn oxidation state, as evident in Fig. 4f . The contribution from Mn 3+ at 641.4 eV in the Mn 2 p 3/2 XPS spectrum significantly increases (from ~5% to 35%) and two additional Mn 2 p 3/2 peaks arise at lower energy (640.4 and 639.4 eV), readily attributable to Mn 2+ . The overall redox process is summarized in Fig. 4g . The presence of thiosulfate was also proven by Fourier transform infrared spectroscopy (FTIR). The FTIR spectrum of Li 2 S 4 ( Supplementary Fig. 6 ) shows an S−S band at 482 cm −1 (ref. 31 ), whereas MnO 2 has a strong antisymmetric MnO 6 stretching vibration at 519 cm −1 (ref. 43 ). The FTIR spectrum of MnO 2 –Li 2 S 4 exhibits a new peak at 670 cm −1 , characteristic of S 2 O 3 2− (ref. 44 ), and one very broad peak at 503 cm −1 midway between the contributions expected from S–S and MnO 2 . We attribute this significant shift of both species to a strong interaction at the interface. To further support the thiosulfate formation mechanism, we investigated the interaction of LiPS with other sulfur hosts—GO (ACS Material, USA) and graphene (ACS Material, single layer). The XPS S2 p spectrum of GO-Li 2 S 4 shows the same components as the MnO 2 –Li 2 S 4 ( Fig. 4c ), which suggests thiosulfate/polythionate surface species are formed here as well. The characteristic peaks are reduced in intensity compared with δ -MnO 2 , as expected. The XPS C 1 s comparison of the GO and GO–Li 2 S 4 confirms the chemical interaction of LiPS in GO–Li 2 S 4 , showing that 20% of the C-O(H) bonds were reduced to C–C (see Supplementary Fig. 7 ). Regarding the S2 p spectrum of graphene–Li 2 S 4 , it shows two contributions at 161.7 and 163.1 eV, identical to that of Li 2 S 4 itself ( Fig. 4d ). This suggests almost no interaction between graphene and polysulfides. The absence of thiosulfate in graphene–Li 2 S 4 implies that the thiosulfate oxygen originates from surface oxy-groups on GO; for MnO 2 , these arise from the OH groups that replace some of the O 2− in the birnessite structure for charge balance. This additional XPS analysis and insight into thiosulfate formation can explain the origin of the excellent cyclability of the MnO 2 nanosheets and that of GO materials [25] , [26] , as discussed in detail below. XPS analysis was further conducted on 75S/MnO 2 nanosheet electrodes extracted from cells at different discharge states ( Fig. 5a–d ). When the cell was discharged to 2.15 V, the presence of long-chain polysulfides is evidenced by strong S2 p 3/2 contributions at 161.7 (S T −1 ) and 162.9 eV (S B −2 ) ( Fig. 5a ) [32] , [39] , with their 1:2 ratio suggesting a chain length approximately equal to Li 2 S 6 owing to the 2:4 ratio of terminal/bridging sulfur in this LiPS. Elemental sulfur was also detected at this and other intermediate states of discharge, consistent with incomplete reaction and/or the disproportionation of metastable polysulfides such as Li 2 S 8 to form Li 2 S 6 and sulfur as previously reported [45] . S2 p peaks between 166 and 170 eV correspond to two sulfur environments: one at 167.2 eV (thiosulfate) and another at 168.2 eV, which is assigned to a polythionate complex as discussed above. These are the same as observed in the S2 p spectrum of MnO 2 –Li 2 S 4 in Fig. 4b . The thiosulfate peak vanishes when the electrode is aged in the coin cell for 20 h after discharge to 2.15 V; only the peak due to the polythionate complex remains in this region. Thus, transformation of thiosulfate to the polythionate complex is accompanied by the conversion of longer-chain polysulfides to shorter-chain polysulfides (~Li 2 S 3 based on the 2:1 ratio of the terminal:bridging sulfur; see Supplementary Fig. 8 , for concentrations of each specific component). Exactly the same reaction is also observed between sodium thiosulfate and polysulfides (Li 2 S 4 ), as shown in Supplementary Fig. 5b . We conclude that S–S from longer-chain polysulfide species reacts with thiosulfate to yield the polythionate complex and shorter polysulfides. Prolonged contact time results in more complete conversion. XPS analysis of the electrode collected at the middle of the second plateau ( Fig. 5c ; 800 mA h g −1 ) shows that the sulfur environments are the same as the electrode discharged to 2.15 V. Their different relative intensities represent the further consumption of longer-chain polysulfides accompanied by the formation of shorter-chain polysulfides. After the electrode was fully discharged to 1.8 V, this process is essentially complete ( Fig. 5d ). The contribution from thiosulfate and the polythionate complex is small, whereas a strong contribution from Li 2 S (S2 p 3/2 at 160.2 eV) along with ~20% Li 2 S 2 (161.7 eV) indicates almost full reduction of sulfur in the electrode. The minority contribution from Li 2 S 2 was assigned based on its very similar binding energy as that of Na 2 S 2 (161.8 eV [32] , and see Supplementary Fig. 9 ). On charge, the XPS spectrum ( Supplementary Fig. 10 ) is similar to Fig. 5a , revealing the re-appearance of the polythionate complex along with polysulfides and sulfur, and indicating that the process is reversible. We propose that the insoluble S 2 O 3 2− that forms on the surface serves as an internal mediator to anchor long-chain polysulfides from solution and trigger conversion to lower polysulfides via the reaction shown below (equation (1)): In this mechanism, the polysulfide catenates to the thiosulfate by insertion in the S–S single bond to create the polythionate complex (I) and a lower polysulfide (that is, Li 2 S 2 or Li 2 S) by an internal disproportionation reaction. This can be explained by the attack of the highly nucleophilic thiosulfate on the bridging S(0) in the polysulfides followed by associative nucleophilic substitution. Sulfur is well known to undergo catenation reactions, such as recently proven for the reaction of sulfur with Li 3 PS 4 to form polysulfidophosphates, Li 3 PS 4+n (ref. 46 ). Elemental sulfur is also susceptible to nucleophilic attack by HS − or SO 3 2− in aqueous solution, resulting in the formation of chains of polysulfides or polythionate complexes, respectively. This is known as the ‘Wackenroder reaction’ [47] . The polythionate complex could also be formed with only one –SO 3 group (equation (2)): However, the bi-polythionate complex (I) is preferred due to its known stability (albeit in aqueous media) [47] . Based on the above model, the electrochemistry of the Li–S system can be explained as follows: (1) initial formation of Li 2 S n (4≤ n ≤8) at the start of discharge gives rise to reaction with MnO 2 , producing thiosulfate at the surface; (2) further reduction produces more polysulfides (4< n <8) that are immediately catenated to form an intermediate polythionate complex and shorter-chain polysulfides ( n <3). The polythionate complex is expected to be poorly soluble, curtailing the polysulfide shuttle. The process occurs progressively on discharge until full conversion to Li 2 S 2 /Li 2 S is achieved. Deposition of lithium sulfide presumably overlays the signature of polythionate complex and thiosulfate, as XPS only probes <10 nm of the surface. To evaluate the efficiency of the thiosulfate mediator, long-term cycling was performed at C/5, C/2 and 2C rates. The two former current densities are suitable for practical applications, while the latter is a benchmark for power utilization. For the C/5 cell ( Fig. 6a ), galvanostatic cycling for over half a year still results in a capacity of 380 mA h g −1 after 1,200 cycles. Similarly good performance was achieved at C/2 ( Fig. 6b ) over 1,500 cycles. After 2,000 cycles at 2C, 245 mA h g −1 useable capacity was still available with good Coulombic efficiency (>98.5%) and a very low decay rate of 0.036% per cycle. The rate was periodically changed to investigate the specific capacity that can be delivered at lower C-rates. After 1,000 cycles at 2C a discharge capacity of 715 mA h g −1 was obtained at C/20, and even after 2,000 cycles at 2C a reversible discharge capacity of 460 mA h g −1 was achieved at C/20 ( Fig. 6c ). The electrochemical robustness extends to cycling at very high C-rates. On switching the C-rate from 3C to C/5, the discharge capacity (985 mA h g −1 ) was 96.3% of the original capacity ( Supplementary Fig. 11 ). At the high rate of 4C, a stable capacity of 700 mA h g −1 was achieved and most of the original capacity was recovered on switching back to a C-rate. Moreover, the overall morphology and structure of the electrode after 1,000 cycles is very similar to that of the original material, as shown in Supplementary Fig. 12 . This suggests that the MnO 2 nanosheet host acts to spatially locate and control both Li 2 S/Li 2 S 2 and sulfur deposition by providing an active interface via the thiosulfate intermediate and demonstrates the excellent stability of this cathode material. 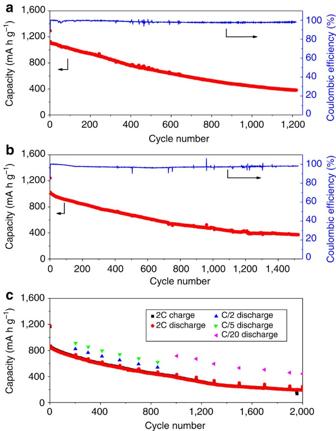Figure 6: Long-term cycling of 75S/MnO2at variable current densities. Capacity and the Coulombic efficiency at (a) C/5 over 1,200 cycles, (b) C/2 over 1,500 cycles, (c) 2C with periodic slow rate for over 2,000 cycles. The capacities of the C/2 and C/5 cells are quite similar to those shown inFig. 2, demonstrating the reproducibility of the electrochemistry. Figure 6: Long-term cycling of 75S/MnO 2 at variable current densities. Capacity and the Coulombic efficiency at ( a ) C/5 over 1,200 cycles, ( b ) C/2 over 1,500 cycles, ( c ) 2C with periodic slow rate for over 2,000 cycles. The capacities of the C/2 and C/5 cells are quite similar to those shown in Fig. 2 , demonstrating the reproducibility of the electrochemistry. Full size image In summary, by the in-situ generation of thiosulfate surface species, which react to form an active complex on the surface of MnO 2 nanosheets, we demonstrate that it is possible to cycle a Li–S cell with a capacity decay as low as 0.036% per cycle over 2,000 cycles, using a classic low viscosity dioxolane (DOL)–dimethyl ether (DME) electrolyte and polyvinylidene fluoride binder. We propose that a new, unique mechanism is responsible, whereby an active polythionate complex serves as an anchor and transfer mediator to inhibit active mass (polysulfide) dissolution into the electrolyte and control the deposition of Li 2 S 2 or Li 2 S. The resultant cells deliver high rechargeable capacity at practical current densities and high sulfur loading. We furthermore note that the thiosulfate mediator is not restricted to support on MnO 2 nanosheets, but is broadly applicable to other support materials and may be also responsible—in whole or in part—for the excellent cycling behaviour observed for GO composites. Unlike previous strategies to trap polysulfides by physical barriers or simple surface interactions, this chemistry is quite efficient. The discovery and understanding of a transfer mediator, which binds polysulfides and promotes stable redox activity, addresses one of the important challenges that face this chemistry. Along with future anticipated improvements in electrolytes and the lithium-negative electrode, this brings the Li–S battery a step closer to practical realization. Preparation of the MnO 2 nanosheets The layered MnO 2 nanosheets were synthesized by a one-step facile method using GO as template. Briefly, 20 mg of single-layer GO (ACS Materials) were dispersed in 100 ml deionized (DI) water by sonication. A well-mixed solution of 10 ml DI water and 160 mg of KMnO 4 (Sigma-Aldrich) was added into the GO suspension and stirred at room temperature for 30 min. The mixture was transferred into a thermostatic oven at 80 °C for 24 h. The resulting material was washed with DI water. Preparation of the 75S/MnO 2 composite For sulfur loading onto the MnO 2 nanosheets, the nano-sized sulfur was first synthesized by reacting 255 mg Na 2 S 2 O 3 (Sigma-Aldrich) with 278 μl concentrated HCl and 17 mg polyvinylpyrrolidone (Sigma-Aldrich) in 85 ml DI water. The MnO 2 nanosheets and nano-sized sulfur were dispersed in 40 ml DI water separately by sonication before being mixed to obtain a homogenous suspension. The suspension was filtered and then dried at 60 °C. The 75S/MnO 2 nanosheet composite was obtained by heating the mixture at 155 °C overnight. Synthesis of Li 2 S 4 Sulfur (Sigma-Aldrich) and Super-Hydride Solution (Aldrich, 1.0 M lithium triethylborohydride in tetrahydrofuran) were mixed together in a 2.75:1 molar ratio until the sulfur was fully dissolved. The resulting solution was dried under vacuum, resulting in precipitation of a yellow powder. A final wash with toluene was conducted, followed by centrifugation to separate the powder from the supernatant to isolate the Li 2 S 4 powder. Preparation of MnO 2 -Li 2 S 4 The MnO 2 nanosheets (87 mg; 1 mmol) were dried at 90 °C under vacuum overnight and dispersed in 10 ml DME solution by sonication in a sealed vial. The mixture was transferred to a glovebox and combined with 10 ml of 0.1 M Li 2 S 4 in DME. The mixture was stirred for 2 h and the product was centrifuged and dried under vacuum overnight. GO-Li 2 S 4 and graphene-Li2S4 samples were prepared by the same procedure. Preparation of MnO 2 -Li 2 S 75S/MnO 2 was mixed with DMF and then cast as a slurry onto a carbon paper current collector. A 2325 coin cell was discharged to 1.8 V at a C/20 rate, using 1 M LiClO 4 in a 1:1 v/v ratio of DOL:DME as the electrolyte with lithium foil as the anode. The cathode was then removed from the coin cell in a glovebox and rinsed with acetonitrile three times before being dried. Electrochemical measurements Cathodes were prepared by casting the DMF slurry containing 75S/MnO 2 nanosheets, 15 wt% Super P carbon and 10 wt % polyvinylidene fluoride onto a carbon paper current collector. Electrochemical studies were carried out using an Arbin cycler in galvanostatic mode, employing electrodes with an average sulfur loading between 0.7 and 1.0 mg cm −2 in 2325 coin cells with lithium foil as the anode and Celgard 3501 separator sheets. Cells were operated in a voltage window of 1.8–3.0 V, except for high-rate studies that were conducted between 1.7 and 3.0 V (2C and 3C rates), and between 1.6 and 3.0 V (4C rate), in an electrolyte comprising 1 M LiTFSI in a 1:1 volume of DME:DOL and 2 wt% LiNO 3 . Specific capacity values were calculated with respect to the mass of sulfur. Electrodes for XPS analysis were prepared by discharging coin cells at C/20 in 1 M LiClO 4 (to avoid sulfur contributions from LiFTSI) in a 1:1 v/v ratio of DOL and DME. Characterization SEM studies were carried out on a Zeiss Ultra field emission SEM instrument and TEM was performed on a Jeol 2010F TEM/STEM operating at 200 KeV. TGA was used to determine the sulfur content of the material, on a TA Instruments SDT Q600 employing a heating rate of 10 °C/min from room temperature to 500 °C under an air flow. FTIR analysis was performed on a Bruker Tensor 37 spectrometer. For XPS, the samples were sealed in a vial before being quickly transferred to the chamber of a ultra-high vacuum Imaging XPS Microprobe system for analysis (Thermo VG Scientific ESCALab 250). All spectra were fitted with Gaussian–Lorentzian functions and a Shirley-type background using CasaXPS software. S2 p peaks were fit using two equal full-width half maximum S2 p doublets with 2:1 area ratios and splittings of 1.2 eV. The binding energy values were all calibrated using the C 1s peak at 285.0 eV. How to cite this article: Liang, X. et al . A highly efficient polysulfide mediator for lithium–sulfur batteries. Nat. Commun. 6:5682 doi: 10.1038/ncomms6682 (2015).